Rapid microbial response to the presence of an ancient relic in the Antarctic Dry Valleys The extreme cold and aridity of the Antarctic McMurdo Dry Valleys have led to the longstanding belief that metabolic rates of soil microbiota are negligible, and that ecosystem changes take place over millennia. Here we report the first direct experimental evidence that soil microbial communities undergo rapid and lasting changes in response to contemporary environmental conditions. Mummified seals, curious natural artifacts found scattered throughout Dry Valleys, alter their underlying soil environment by stabilizing temperatures, elevating relative humidity and reducing ultraviolet exposure. In a unique, multi-year mummified seal transplantation experiment, we found that endemic Dry Valley microbial communities responded to these changes within 3 years, resulting in a sevenfold increase in CO 2 flux and a significant reduction in biodiversity. These findings challenge prevailing ideas about Antarctic Dry Valley ecosystems and indicate that current and future environmental conditions may strongly influence the ecology of the dominant biota in the Dry Valleys. Since Scott's 1901–1904 Discovery expedition, mummified seals have been reported in the McMurdo Dry Valleys of Antarctica in locations up to 66 km inland and 1,800 m above sea level [1] , [2] , [3] , [4] , [5] , [6] , [7] . These curious, twisted remnants of bone and desiccated flesh ( Fig. 1a ) are many hundreds of years old, preserved by extremely cold and arid conditions [1] , [2] , [5] , [6] . Why they journey over such challenging terrain to arrive at these remote resting places is unknown and has generated much speculation [2] , [4] , [5] , and theories have ranged from the random dispersal of disoriented pups during prolonged bad weather [2] to outbreaks of phocine distemper virus [6] . Meanwhile, the ecological significance of the phenomenon has remained unexplored. 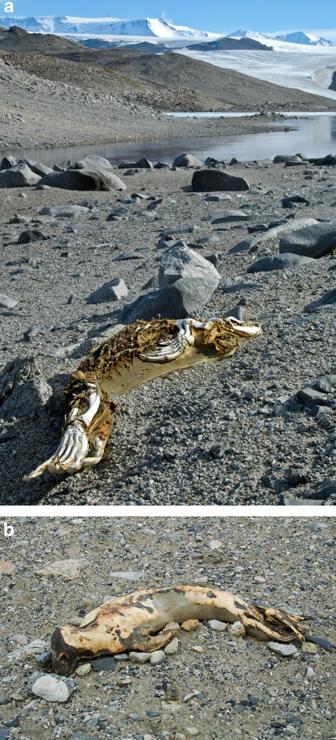Figure 1: Mummified seal carcasses in the Miers Valley. (a) A seal carcass in a stage of advanced mummification. (b) The mummified seal carcass used for the seal movement experiment. Figure 1: Mummified seal carcasses in the Miers Valley. ( a ) A seal carcass in a stage of advanced mummification. ( b ) The mummified seal carcass used for the seal movement experiment. Full size image The Dry Valleys comprise one of the most inhospitable, trophically simple ecosystems on Earth [8] , [9] . Devoid of vascular plant life [8] , [9] , [10] , the Dry Valley ecosystem supports only a handful of microscopic invertebrate, lichen and moss species [9] , [10] . However, the bulk of Dry Valley biodiversity and biomass consists of edaphic bacteria [8] , [11] , [12] , as few other organisms can endure the region's extreme temperature and light regimes, high soil salt concentrations, near-negligible levels of organic C and N, and scarcity of liquid water [10] , [12] . It has been suggested that these soil microbial communities are principally sustained and structured by the location and distribution of legacy C sources in the form of ancient lake sediments [13] , [14] , [15] , [16] . Under this hypothesis, contemporary environmental conditions exert limited influence on community dynamics [13] , [15] , as microbial activity in the Dry Valleys has, until recently, been thought to be exceptionally low compared with temperate ecosystems [13] , [15] . Activity is further restricted to brief periods during austral summers, when liquid water may be available in certain niche habitats [17] , [18] , [19] . As a result, changes in soil ecology are believed to take place over centuries and even millennia [13] , [15] , despite the fact that no direct studies have been conducted on rates of change in microbial community structure and function. Instead, researchers studying Dry Valley soil ecosystems have used CO 2 efflux and rates of organic C turnover in soil as proxies for microbial activity, and as low activity rates ipso facto preclude changes in community structure, data showing low rates have been taken to indicate slow rates of change in microbial communities. For example, Johnston and Vestal's study of Dry Valley cryptoendoliths [20] used the slow lipid C turnover rate ( ∼ 20,000 years) to support the claim that they are the slowest-growing communities on earth. Therefore, despite widespread acknowledgment of the susceptibility of Dry Valley microbial communities to seasonal variations in biological activity [15] , [21] , [22] , [23] , no study has described or predicted rapid and sustained changes in community structures caused by contemporary environmental conditions. More recent studies have shown that the Dry Valleys support a phylogenetically diverse group of microbes [12] , [24] , [25] , and a handful of these studies have speculated that these communities respond on much shorter, decadal timescales [15] , [19] , [21] , [26] . In this study we have compared soil beneath a seal carcass found in the Miers Valley, Victoria Land, Antarctica, with soils from nearby exposed control sites to characterize the physicochemical and biological modifications associated with the mummified seal. We measured the rate at which the observed biological changes occurred in response to a direct soil modification experiment: after transplanting a Miers Valley mummified seal to an untouched neighbouring site, we used community DNA fingerprinting and amplicon pyrosequencing over several years to track changes in microbial community composition and structure. Our observations in the soil modification experiment confirm the view that microbial communities can respond to changes in the environment, offering the first direct evidence of rapid microbial response to contemporary environmental conditions in the Dry Valleys. Radiocarbon ages of mummified seals Mummified seals found within the McMurdo Dry Valleys seem to range widely in age, as indicated by radiocarbon dating data of the tissues from a number of seals in Miers Valley (including the seal, 'Seal I', used for the movement experiment; Table 1 ; Supplementary Methods ). Radiocarbon dating of Antarctic marine fauna is complicated by the marine reservoir effect, which results from the unusual radiocarbon content of Southern Ocean coastal waters. These waters originate from deep currents that have travelled for millennia along the seafloor, carrying ancient dissolved atmospheric CO 2 . The 14 C-depleted CO 2 then enters the food chain and leads to significant overestimation of radiocarbon age for top-level feeders in the Southern Ocean [2] , [27] . To help correct age estimates for the mummy tissue, a tissue sample taken from a seal carcass killed during Scott's 1904 expedition and left outside the Cape Evans hut was dated and used for calibration ( Table 1 ). Mummified seals in this small set of samples were estimated to be around 250–790 years old ( Table 1 ), and are evidently enduring features of the Dry Valley landscape and ecosystem. Table 1 Radiocarbon dating of seal tissue samples near Miers Valley. Full size table Long-term changes beneath a mummified seal Physicochemical comparison of soil beneath an untouched mummified seal carcass in Miers Valley ( Fig. 1b ) with soil from a nearby exposed control site of similar geomorphology revealed substantial modifications. 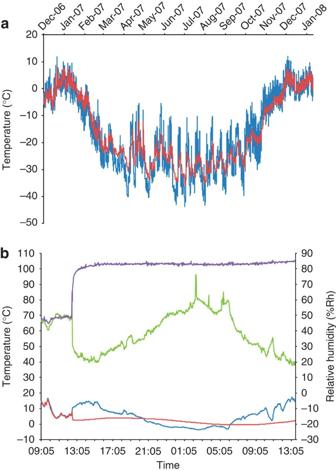Figure 2: Soil temperature and relative humidity beneath and adjacent to a seal carcass. (a) Temperatures beneath (red, mean=−16.1±12.3 °C) and adjacent to (blue, mean=−16.5±13.8 °C) the moved seal carcass in Miers Valley, from December 2006 to January 2008, measured every 30 min (total of 16,240 measurements). (b) Relative humidity beneath (purple, mean=82.8±1.8% Rh) and adjacent to (green, mean=37.7±13.1% Rh) the carcass. Temperature measurements beneath (red, mean=1.8±1.6 °C) and adjacent to (blue, mean=4.7±5.9 °C) the carcass were taken simultaneously with the relative humidity measurements. Measurements were made 10–11 December 2006 at 2-min intervals (total of 920 measurements). Means are given with ±1 s.d. Soil N and organic C levels under the seal were elevated to nearly 7× and 4× the levels in controls, respectively ( Table 2 ), suggesting that large quantities of seal organic matter were transferred to the soil over time. Analysis of the isotopic N composition of seal tissue and seal-covered soil lends further support to this conclusion: Dry Valley materials typically have very low fractions of 15 N, whereas seal tissue and seal-covered soil both yielded high 15 N fractions characteristic of Antarctic marine-derived materials ( Supplementary Table S1 ). Differences in total C levels between seal-covered and unaugmented control soils were highly significant ( t =7.754687, P <0.0001, n =4 and 6; unpaired two-tailed t -test). Total N and total organic C levels were likewise significantly different between the two sites ( t =7.808302, P <0.0001, n =4 and 6; t =7.432392, P <0.0001, n =4 and 6 for total N and total organic C, respectively; unpaired two-tailed t -test). Table 2 Soil augmentation by seal carcass. Full size table The presence of the seal carcass appeared to stabilize considerably the extreme diurnal temperature fluctuations in the soil ( F =1.26091, P <0.00001, n =16,240; two-tailed F -test for variances, Fig. 2 ), yet had little influence on the average temperature (−16.1±12.3 °C for seal-covered soil versus −16.5±13.8 °C for control site, Fig. 2 ). More importantly, soil beneath the carcass experienced significantly elevated and stabilized relative humidity levels (82.8±1.8% for seal-covered soil versus 37.7±13.1% for control site, Fig. 2 ). These physicochemical differences were accompanied by marked differences in resident microbial communities ( Table 2 ). Average bacterial cell counts of seal-covered samples were an order of magnitude higher than those of control sites ( t =14.35, P <0.0001, n =8 and 9; unpaired two-tailed t -test), average CO 2 flux was significantly greater ( t =5.109235, P <0.0001, n =12 and 16; unpaired two-tailed t -test) and adenosine triphosphate (ATP) levels (a proxy for microbial biomass and activity) were higher by a factor of 25 ( t =4.241930, P =0.0017, n =6; unpaired two-tailed t -test). Figure 2: Soil temperature and relative humidity beneath and adjacent to a seal carcass. ( a ) Temperatures beneath (red, mean=−16.1±12.3 °C) and adjacent to (blue, mean=−16.5±13.8 °C) the moved seal carcass in Miers Valley, from December 2006 to January 2008, measured every 30 min (total of 16,240 measurements). ( b ) Relative humidity beneath (purple, mean=82.8±1.8% Rh) and adjacent to (green, mean=37.7±13.1% Rh) the carcass. Temperature measurements beneath (red, mean=1.8±1.6 °C) and adjacent to (blue, mean=4.7±5.9 °C) the carcass were taken simultaneously with the relative humidity measurements. Measurements were made 10–11 December 2006 at 2-min intervals (total of 920 measurements). Means are given with ±1 s.d. Full size image Changes in bacterial diversity beneath a mummified seal Ultra-deep pyrosequencing (>30,000 reads per sample, average length 369.5 bp) of bacterial 16S rRNA gene PCR amplicons revealed a significant shift in microbial community structure and a reduction in apparent diversity in seal-covered soil relative to control soil ( Fig. 3a,b ), based on operational taxonomic units (OTUs 0.03 ) defined at 97% similarity. The seal-covered ( Fig. 3b ) site supported significant populations of only two of the seven most abundant phyla observed in the control site ( Fig. 3a ), Actinobacteria and Bacteroidetes. It was dominated by two OTUs 0.03 —one assigned to a Psychrobacter sp. (γ-proteobacteria, accounting for 34.3% of reads), and one affiliated with the Planococcaceae family (Firmicutes; 24.2% of reads)—that were <0.5% abundant in control soil. Furthermore, the top nine most abundant OTUs 0.03 in the control sample, comprising ∼ 36% of all reads, were all found in the seal-covered sample at the considerably reduced abundance of ∼ 2% of total reads. Finally, the reduction in apparent microbial diversity is reflected in the numbers of OTUs 0.03 at >1% abundance, which decreased from 26 in the control sample to 11 in the seal-covered sample. 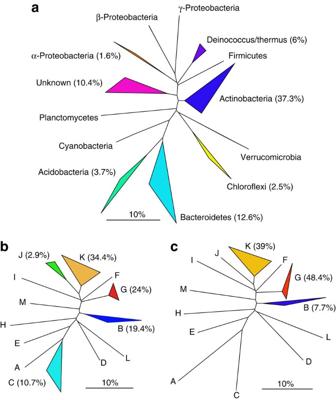Figure 3: Phylum-level diversity of bacterial 16S rRNA gene sequences from soil sites. Percentage abundance of phyla within each site are shown (in parentheses) for the (a) exposed control site, (b) original seal-covered site and (c) new seal-covered site. Unnumbered branches are <1% but >0%. 454 pyrosequencing reads were denoised and clustered at 97% (furthest neighbour) to obtain 1,062 operational taxonomic units (OTUs0.03) in total, of which 261 OTUs0.03were shared. The sample for (a) was collected in January 2005; sample (b) in January 2007; and sample (c) in January 2009. Figure 3: Phylum-level diversity of bacterial 16S rRNA gene sequences from soil sites. Percentage abundance of phyla within each site are shown (in parentheses) for the ( a ) exposed control site, ( b ) original seal-covered site and ( c ) new seal-covered site. Unnumbered branches are <1% but >0%. 454 pyrosequencing reads were denoised and clustered at 97% (furthest neighbour) to obtain 1,062 operational taxonomic units (OTUs 0.03 ) in total, of which 261 OTUs 0.03 were shared. The sample for ( a ) was collected in January 2005; sample ( b ) in January 2007; and sample ( c ) in January 2009. Full size image The seal transplant experiment In light of the differences we observed in microbial community structure between seal-covered and control soils, we devised a unique, controlled, long-term soil modification experiment to investigate how quickly these changes occurred. A 250-year-old mummified Miers Valley seal carcass (Seal I in Table 1 ) was transplanted to an exposed pristine location of similar geomorphology during the 2005–2006 austral summer, and soil samples were collected from the carcass's original location ('original site'), the new location ('new site') and control sites at zero-time and for four succeeding austral summers. Total DNA was extracted from the samples for community profiling and structure comparisons. Using two distinct microbial community DNA fingerprinting techniques, automated ribosomal intergenic spacer analysis (ARISA) and terminal restriction fragment length polymorphism (tRFLP), rrn operon-based profiles were generated for the bacterial communities in each sample. When subjected to multidimensional scaling analysis, both the ARISA and the tRFLP community profiles showed that within only two summers after introducing the seal carcass, 'new site' soil bacterial communities directly in contact with the carcass abdomen resembled those of the 'original site' ( Fig. 4 ), where the seal had resided for over 250 years (Seal I in Table 1 ). Only soils underneath the abdomen were in direct contact with the seal carcass, which arched upward as mummification progressed. The Y0 zero-time samples for the 'new site', which collectively cover a 25-m 2 area, group closely with control samples taken in subsequent years, indicating that the 'new site' is microbiologically representative of the surrounding area before the introduction of the seal carcass. Profiling results for fungal communities showed similar trends ( Supplementary Fig. S1a ), but the photoautotrophic cyanobacterial communities did not exhibit conclusive patterns ( Supplementary Fig. S1b ). 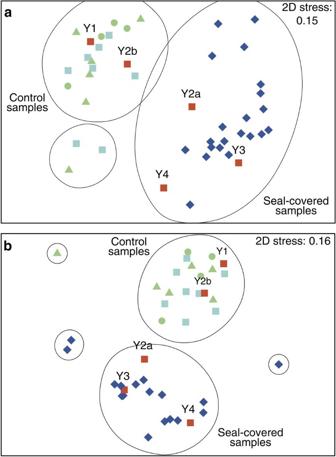Figure 4: Genotyping analyses of bacterial communities. Bacterial ARISA (a) and tRFLP (b) profiles for samples taken from control (Y0: green circles; Y1–Y4: green triangles), original seal-covered (blue diamonds) and new seal-covered sites (non-contact: cyan squares; contact: red squares, with labels indicating year of sampling) were analysed and presented on multidimensional scaling (MDS) plots. Thresholds of similarity are represented by solid contours at 20 and 30% for ARISA and tRFLP, respectively. The two-dimensional (2D) stress values indicate that the plots are reasonable representations of distances between samples. Figure 4: Genotyping analyses of bacterial communities. Bacterial ARISA ( a ) and tRFLP ( b ) profiles for samples taken from control (Y0: green circles; Y1–Y4: green triangles), original seal-covered (blue diamonds) and new seal-covered sites (non-contact: cyan squares; contact: red squares, with labels indicating year of sampling) were analysed and presented on multidimensional scaling (MDS) plots. Thresholds of similarity are represented by solid contours at 20 and 30% for ARISA and tRFLP, respectively. The two-dimensional (2D) stress values indicate that the plots are reasonable representations of distances between samples. Full size image Soil bacteria cell counts were also carried out for the seal movement experiment ( Fig. 5 ; Supplementary Methods ). When the seal carcass was moved in Y0, bacterial cell counts of established 'original site' samples indicate microbial biomass one order of magnitude higher than control sites ( Table 2 ); the same is true for the year prior (Y[−1]) ( Fig. 5 ). With the seal carcass in its new place after Y0, overall 'new site' sample cell counts remained statistically indistinguishable from those of control sites for the entirety of the experiment, except 'new site' samples in Y3 that experienced direct contact with the seal abdomen, which exhibited an increase in microbial biomass ( Fig. 5 ). A two-way analysis of variance of average cell counts during Y1–Y3 showed significant interaction between site and year factors ( F =14.63, P <0.0001, d.f.=6), with site effects accounting for 27% of variance ( F =21.87, P <0.0001, d.f.=3) and time effects accounting for only 4% of variance ( F =4.47, P =0.0143, d.f.=2). Intriguingly, the 'original site' microbial biomass declined rapidly after the seal was moved, even though the composition of these communities, based on DNA profiling results, remained stable over time ( Fig. 4 ). 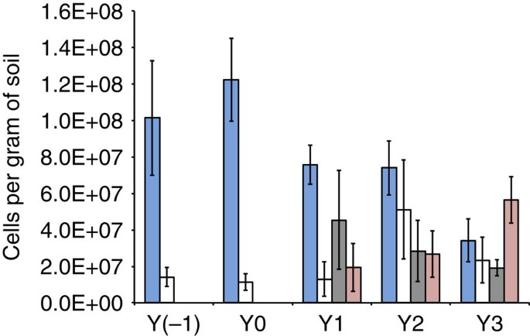Figure 5: Soil bacterial direct cell counts for seal movement experiment. Direct bacterial cell counts for samples taken from the old seal-covered site (blue), control sites (white), the new seal-covered site (gray) and the new seal-covered site samples in direct contact with the seal abdomen (red). Averages were calculated from ten measurements on the same sample with top and bottom outliers excluded (n=8), and error bars indicate ±1 s.d. Figure 5: Soil bacterial direct cell counts for seal movement experiment. Direct bacterial cell counts for samples taken from the old seal-covered site (blue), control sites (white), the new seal-covered site (gray) and the new seal-covered site samples in direct contact with the seal abdomen (red). Averages were calculated from ten measurements on the same sample with top and bottom outliers excluded ( n =8), and error bars indicate ±1 s.d. Full size image Amplicon pyrosequencing analysis of the altered 'new site' community provided a more detailed view of the rapid changes in community structure. The 'new site' community ( Fig. 3c ) exhibited a shift in microbial communities similar to that observed in the 'original site' seal-covered community ( Fig. 3b ) through ARISA and tRFLP community fingerprinting ( Fig. 4 ). In fact, the same two OTUs 0.03 affiliated with Psychrobacter sp. (γ-proteobacteria) and the Planococcaceae family (Firmicutes) in the 'original site' seal-covered sample dominated the 'new site' community to an even greater extent, constituting over 85% of observed sequences (38.9 and 47.5%, respectively), and the 'new site' community was dominated by only three of the five most abundant phyla observed in the already less diverse 'original site' community. Bacteroidetes, which was abundant in both the control and 'original site' samples, was present at <1% in the 'new site' sample. Although various biases may affect the quantitativeness of amplicon pyrosequencing analysis, they are unlikely to account for the drastic shifts in apparent diversity reported here. Notably, none of the newly dominant OTUs 0.03 seem to have been introduced by the seal carcass, as they were all observed in the control sample, albeit at very low abundances ( ∼ 2% of reads) ( Supplementary Fig. S2 ). It would appear that changes in microbial ecology associated with the presence of the carcass resulted from differential responses of indigenous organisms. Indeed, the 20 overall most abundant phylotypes ( ∼ 80% of all sequences) were found in all three sites (at read numbers ranging from 2 to 27,691, Supplementary Table S2 ), indicating that microorganisms exclusively associated with the seal carcass exert relatively little, if any, influence on the microbial ecology of surrounding habitats. Therefore, the short-term impact of carcass presence was manifested in a rapid increase in the dominance of a small group of organisms at the expense of nearly all of the previously abundant indigenous taxa. This resulted in a substantial shift in microbial community structure, loss of apparent biodiversity and a 2.4× increase ( P =0.0018, n =9; unpaired one-tailed t -test) in microbial biomass relative to the control samples in Y3 ( Fig. 5 ). The influence of abiotic factors on soil microbial communities The seal carcass produced specific physicochemical changes in underlying soil ( Table 2 ). Although differences in elemental composition of 'original site' and control site soils, which is reflective of the underlying soil geomorphology, were not significant ( t= 0.5461512, d.f.=29, P =0.5891, n =3 and &6; paired two-tailed t -test), there were significant differences in pH (pH 8.03±0.60 for 'original site' versus pH 10.16±0.18 for control sites; t =6.749925, P <0.0001, n =4 and 8; unpaired two-tailed t -test). Conductivity also differed significantly between sites (1,048±395 μS cm −1 for 'original site' versus 455±163 μS cm −1 for control sites; t= 2.828623, P =0.0179, n =4 and 8; unpaired two-tailed t -test). To determine which sets of physicochemical parameters might best explain differences in community DNA fingerprinting profiles, five representative samples were subject to BEST (Biota-Environment STepwise matching) analysis (PRIMER 6). Variables examined included average pH; average conductivity; percent weight of total N, C and organic C; and mass concentrations of Li, B, Na, Mg, Al, Si, P, S, K, Ca, V, Cr, Fe, Mn, Co, Ni, Cu, Zn, As, Se, Sr, Ag, Cd, In, Ba, Hg, Pb, Bi and U. For all sets of five variables or fewer, the global sample statistic was ρ =0.527 with a significance level of 71% (out of 99 random permutations). The low ρ -value and high significance level of the global sample statistic indicate that the variables we examined do not account satisfactorily for the differences in community DNA fingerprinting profile and, by extension, bacterial community composition over time. This is an interesting result, given that the differences in total C, total N, organic C, pH and conductivity between 'original sites' and control sites were demonstrably significant ( Table 2 ). It is possible that bulk augmentation of organic C alone has little effect on community structure, while specific organic compounds, present at concentrations below detection limit, do. The seal carcass may also supply additional compounds that chelate nutrients in the soil, making them more biologically available to resident microbes. However, changes in bacterial community composition ( Fig. 4 ) do appear to precede significant increases in microbial biomass ( Fig. 5 ), suggesting that variables other than nutrient input from the seal carcass, such as reduced temperature fluctuation, increased relative humidity and reduced ultraviolet exposure, may have significant roles in determining bacterial diversity in Dry Valley soils. Indeed, cell counts from the 'original site' showed rapid decline after the seal movement, despite persistently elevated levels of soil C and N ( Fig. 5 ), suggesting that physical changes enacted by a carcass, and not nutrient supplementation, have the most profound effect on microbial community composition. Our results show that significant changes in the structure of Antarctic soil microbial communities associated with the presence of a seal carcass can take place within a few years under favourable conditions, and these changes seem to dramatically reduce biodiversity. These findings complement previous indirect estimates of organic C turnover in the Dry Valleys [15] , [19] , [21] , [22] , [23] , [26] , and provide the first direct experimental evidence that the surprisingly rapid turnover rate can influence the ecology of the dominant biota in the Dry Valleys. Because of strict regulations on performing manipulative experiments in the Dry Valleys, our observations were based on results from transplanting a single mummified seal carcass. However, few manipulative experiments of any sort have been performed in situ in the Dry Valleys [19] , [28] , which in part accounts for the unexpected character of our results. In particular, differences in community DNA fingerprinting profiles failed to correlate with the chemical properties of their respective soils. It seems that abiotic physical modifications associated with the presence of a seal carcass, rather than nutrient or biological inputs, led to the observed changes in microbial communities. This hypothesis is counter-intuitive and requires further experimental validation (for example, by placing a large and heavy object on an untouched patch of Dry Valley soil and performing similar measurements); however, should it be proven correct, it could mean that the transformational effect of the mummified seal carcass may be mimicked in other Dry Valley soils associated with other landscape features capable of effecting similar abiotic modifications, such as boulders and large rocks. Thus a significant portion of Dry Valley microbiota in soils around boulders and large rocks may be at least partially responsive to contemporary conditions rather than primarily to legacy resource inputs, as widely believed [13] , [15] , [22] . It has been shown in more complex ecosystems that decreases in biodiversity alter ecosystem function [29] which, for the Dry Valleys, remains largely unknown [12] . Our data show that, with moderate changes in physical conditions, the microbiota in Dry Valley soils can respond within timeframes considerably shorter than centuries or millennia. Therefore, loss of microbial diversity and functional adaptation of the Dry Valley ecosystem in response to climatic changes may occur much more rapidly than has been suggested [15] , [21] , [30] . Such prediction is consistent with the current view that Antarctic soils are inherently sensitive to climate variability, as minor temperature variations can lead to cascading changes in hydrology and biogeochemical cycling, which will potentially affect ecosystem processes [15] . Any change in climatic conditions will be accompanied by multiple environmental stressors, including modifications in temperature, water availability and nutrients. Our findings show that indigenous microbial communities of Dry Valley soils can experience rapid and sustained structural alterations in response to contemporary variance in environmental conditions. Because the communities examined do not reside in areas where rapid response might be expected—such as streambeds [28] , lakeshores [19] and other hyporheic zones—this unexpected sensitivity to environmental disturbance is all the more striking, and may in fact characterize a substantial and previously unsuspected portion of Dry Valley microbiota. Seal movement experiment On 30 January 2006, a mummified crabeater seal was carried from its original resting site near Lake Miers (S 78°05′36″, E 163°51′22″), Miers Valley, Victoria Land, Antarctica, to a new site of similar geomorphology 20 m north. Soil samples (>10 g each) were collected aseptically from a depth range of 0–5 cm during the austral summers 2004–2005 (Y[−1]), 2005–2006 (Y0), 2006–2007 (Y1), 2007–2008 (Y2), 2008–2009 (Y3) and 2009–2010 (Y4). Samples from the original site for years Y[−1] to Y4 were collected from areas where the mummy head, abdomen and tail had rested. Corresponding new site samples were collected from beneath the seal in Y1–Y4, with Y0 samples taken along two 5-m crossing transects before the seal was moved into place. Controls in all years were collected at a distance >10 m away from the seal. Samples were stored in sterile plastic containers at −80 °C until analysis. Physicochemical and biological activity measurements For copy number analysis, soil samples (2 g) were finely ground with an agate mortar and pestle. Total C and total N were determined by combusting 250 mg of powder in a Leco TruSpec CN analyzer (LECO Corp., St Joseph, MN, USA) at the University of Waikato Stable Isotope Laboratory. For total organic C, fractions of ground sample (1 g) were acidified with excess 1 M H 2 PO 4 to remove carbonates, digested overnight at 37 °C, and neutralized with 3 M NaOH. After drying, samples were massed and combusted as described above. pH and conductivity were determined using the slurry technique with a mass ratio of 2:5 sample to deionized water. Samples for spectrochemical element analysis were air-dried and digested with HCl and HNO 3 according to US EPA Analytical Method 200.2 (Revision 2.8, 1994). A procedural blank containing no soil was included. Samples were then analysed using a Perkin-Elmer SciEX ELAN DRC II ICP-MS (GE Healthcare). All samples were mixed 1:1 with an internal standard (2 p.p.m. Sc, 2 p.p.m. Ga, 200 p.p.b. Te, 40 p.p.b. Rh, 20 p.p.b. Lu and 2% HNO 3 ) to correct for drift. Temperature and relative humidity recordings were taken every 2 min for 25 h from 10–11 December 2006 using iButton temperature and relative humidity loggers (model DS1923; Maxim Integrated Products, Sunnyvale, CA, USA) placed at a 2-cm depth under the seal abdomen and at a 50-cm distance from the seal extremity. Long-term temperature readings were taken every 36 min from December 2006 to January 2008 using a HOBO datalogger (Onset Computer Corp., Bourne, MA, USA) with probes placed under the seal abdomen and at an adjacent exposed location. ATP abundances were measured in triplicate by mixing 100 mg of soil samples with 100 μl of extractant buffer (Bev-Trace, 3M-Biotrace, Brigend, UK), which were incubated for 1 min before 75 μl of reconstituted luciferase was added. ATP abundance was determined using an ATP luminometer (Uni-Lite, 3M-Biotrace). Soil CO 2 flux was measured in the field with a portable infrared gas analyzer (LiCor 6400 Portable Photosynthesis System with 6400-09 soil CO 2 flux chamber, LiCor Inc., Lincoln, NE, USA). Four PVC soil collars were inserted to a depth of 6 cm at each site and remained in place throughout the experiment, minimizing disturbance while enabling repeated measurements of CO 2 flux from the same soil surface. The closed gas exchange system was customized to measure small changes in chamber CO 2 concentrations following efflux from soil [31] . Soil temperature at 5-cm depth was measured every 6 s during the 20-min gas measurement period using the LiCor system temperature probe along with several HOBO outdoor temperature loggers (Onset Computer Corp.). The loggers were placed at 5-cm depth and were evenly spaced throughout the four replicate soil collars to provide an average temperature across the site. Bacterial community fingerprinting using ARISA and tRFLP DNA was extracted from soil samples using a modified version of a previously published CTAB (cetyltrimethylammonium bromide) bead-beating protocol [32] and quantified using the Quant-IT dsDNA BR Assay Kit (Invitrogen, Carlsbad, CA, USA). PCRs were performed in triplicate and pooled to reduce stochastic inter-reaction variability between runs [33] . Each 25-μl ARISA reaction (30 μl, tRFLP) contained 10 ng extracted community DNA, 1-U Platinum Taq DNA polymerase (1.5 U for tRFLP), 1× Platinum Taq PCR buffer (Invitrogen Ltd., New Zealand), 0.2 mM dNTPs, 1.5 mM MgCl 2 (2.5 mM for tRFLP), 0.02 mg ml −1 BSA (0 mg ml −1 for tRFLP), 0.75 μM each of forward and reverse primer (0.4 μM for tRFLP) and PCR-grade water. Before template DNA was added, PCR master mixes were treated with ethidium monoazide to inhibit potential contaminating DNA [34] . PCR primers for bacterial ARISA were ITSF (5′-GTCGTAACAAGGTAGCCGTA-3′) and ITSReub (5′-HEX-GCCAAGGCATCCACC-3′) [35] . Thermal cycling conditions were 94 °C for 2 min; 30 cycles of 94 °C for 45 s, 55 °C for 30 s and 72 °C for 2 min; and 72 °C for 7 min. After cycling, reactions were pooled and purified using a QuickClean 5 M PCR Purification Kit (GenScript Corp., USA). Bacterial tRFLP PCR primers were 787F (5′-FAM-ATTAGAWACCCBGGTAGTC-3′), a truncated version of Tx9 and 1391R (ref. 36 ), designed to amplify the same hypervariable region as the 454-pyrosequencing analysis. Thermal cycling conditions were 94 °C for 3 min; 30 cycles of 94 °C for 20 s, 53 °C for 20 s and 72 °C for 45 s; 72 °C for 3 min. Reactions were electrophoresed and size-selected using a QuickClean DNA Gel Extraction Kit (GenScript Corp., USA). In reaction volumes of 20 μl, 400 ng of community DNA were digested with 2-U Msp I and 1× restriction enzyme buffer (Roche Applied Science, Indianapolis, IN, USA) at 37 °C for 5 h and terminated at 65 °C for 20 min. See Supplementary Methods for information on fungal and cyanobacterial community fingerprinting. Lengths of fluorescent-labelled tRFLP and ARISA fragments were determined by capillary electrophoresis using an ABI 3130 Genetic Analyzer at 10 kV and a separation temperature of 44 °C for 2 h. The resulting fragment profiles were exported in PeakScanner using the minimal 5 RFU cutoff. A noise level was calculated from the data, and only peaks whose amplitude exceed three times the standard deviation of the noise were retained [37] . The remaining peaks were then size-binned, clustered and normalized to relative abundance data [37] . Fragment length abundances for each sample were imported into PRIMER 6 software (v.6.1.6; PRIMER-E, Plymouth, UK 2006), converted to presence/absence data, and used to calculate Sørensen similarities (one minus Bray-Curtis dissimilarity) across samples. To visualize the results, non-metric multidimensional scaling was performed with 100 iterations of bootstrapping. Agglomerative, hierarchical clustering of similarities was performed using the CLUSTER method, and this information was superimposed on the plots to create contours designating thresholds of similarity. 454-Pyrosequencing of PCR amplicons PCR amplicons containing the V5–V7 hypervariable regions of bacterial 16S rRNA gene were generated for the original (Y[−1]), control (Y1) and new (Y3) sites using the primer pair Tx9 (5′-GGATTAGAWACCCBGGTAGTC-3′) and 1391R (5′-GACGGGCRGTGWGTRCA-3′) [36] . PCR was performed in triplicate and pooled to reduce stochastic variability between reactions [33] . Each 30 μl reaction contained 5 or 20 ng of extracted community DNA, Pfx polymerase and platinum polymerase (0.5 U each; Invitrogen), 1× Pfx PCR buffer with Pfx enhancer, 0.2 mM dNTPs, 1 mM MgCl 2 , 0.02 mg ml −1 BSA, 0.8 μM of forward and reverse primer, and PCR-grade water. Thermal cycling conditions were 94 °C for 2 min; 18 or 24 cycles of 94 °C for 15 s, 55 °C for 30 s and 68 °C for 1 min; and 68 °C for 3 min. Amplicons were size-selected and purified using polyacrylamide gel electrophoresis before being prepared for pyrosequencing by Taxon Biosciences (Tiburon, CA, USA). The denoised 16S rRNA gene amplicon sequences have been deposited in GenBank under accession codes HM990023 to HM990100 . Original pyrosequencing flowgram files are available from the Sequence Read Archive ( http://www.ebi.ac.uk/ena/data/view/ERP001015 ). Analysis of pyrosequencing data Pyrosequencing flowgrams (that is, sff files) were filtered and denoised using a variation of the AmpliconNoise suite [38] adopted for FLX Titanium sequences. Reads that had at least one flow with signal intensity between 0.5 and 0.7 or a cycle of four nucleotide flows (TACG) that failed to give a signal >0.5 before cycle #400 (both indicative of noise) were discarded, and all reads were truncated at cycle #600. Pyrosequencing noise was removed using PyroNoise [38] using the default settings, and PCR noise was removed using SeqNoise [38] ( σ s =0.033, c s =0.08) after truncation at 400 bp to reduce noise further. Finally, the sequences were checked for PCR chimeras using Perseus [38] ( α =−7.5, β =0.5). The resulting sequences were aligned with prank+F (ref. 39 ), then analysed using Mothur (version 1.11.0) [40] . OTU 0.03 (furthest neighbour at 97% similarity) representative sequences were classified using the RDP Classifier [41] . Phylogenetic analysis of sequences was performed with representative sequences of the top 78 OTUs 0.03 (>0.1% overall abundance in pyrosequencing data sets, representing 145,580 reads). Taxonomic trees were constructed using ARB [42] , with DNADIST and neighbour joining analysis. Statistical analyses To determine which subset of environmental parameters might best explain differences in ARISA fragment profiles, physicochemical and fragment-profile data for five representative samples (two seal-covered samples from Y[−1] and Y0, and three control samples from Y[−1], Y0 and Y2) were imported into PRIMER 6 software for BEST analysis [43] . BEST calculates the value of Spearman's rank correlation coefficient ( ρ ) using every possible combination of variables until it finds the subset, whose Euclidean distance matrix gives the highest value ρ ('best' match) for a given resemblance matrix. The fragment profile resemblance matrix was calculated using the S 17 Bray-Curtis similarity coefficient. For statistical tests performed throughout the study, all data were checked to satisfy underlying assumptions of the tests applied. All differences in n between analyses were due to availability of soil material, which was limited. Accession codes: The processed 16S rRNA gene amplicon sequences have been deposited in GenBank Nucleotide Core Database under accession codes HM990023 to HM990100 . How to cite this article: Tiao, G. et al . Rapid microbial response to the presence of an ancient relic in the Antarctic Dry Valleys. Nat. Commun. 3:660 doi: 10.1038/ncomms1645 (2012).